Bulk mixed ion electron conduction in amorphous gallium oxide causes memristive behaviour In thin films of mixed ionic electronic conductors sandwiched by two ion-blocking electrodes, the homogeneous migration of ions and their polarization will modify the electronic carrier distribution across the conductor, thereby enabling homogeneous resistive switching. Here we report non-filamentary memristive switching based on the bulk oxide ion conductivity of amorphous GaO x ( x ~1.1) thin films. We directly observe reversible enrichment and depletion of oxygen ions at the blocking electrodes responding to the bias polarity by using photoemission and transmission electron microscopies, thus proving that oxygen ion mobility at room temperature causes memristive behaviour. The shape of the hysteresis I-V curves is tunable by the bias history, ranging from narrow counter figure-eight loops to wide hysteresis, triangle loops as found in the mathematically derived memristor model. This dynamical behaviour can be attributed to the coupled ion drift and diffusion motion and the oxygen concentration profile acting as a state function of the memristor. A memristor is a resistive switching device that varies its internal resistance state according to the history of the applied voltage and current [1] , [2] , [3] . Following the definition by Chua et al. [1] , [2] , it can be described by a set of equations including the current equation, V = R ( w , I ) I , and a rate equation, d w /d t = f ( w, V ). Here V , I and R are the voltage, current and resistance, respectively. w is an internal state variable, described by a time-varying function f , and it is crucial to the switching dynamics of the memristor. The time-dependent switching suggests that a memristor could be a physical system that enables to emulate the synaptic memory function more directly than the complementary metal-oxide semiconductor system [4] , [5] , [6] , [7] . Recently, memristive resistive switching of many transition metal-oxide-based semiconductor films has been extensively studied [4] , [8] , [9] , [10] . The formation [9] , [10] , [11] , [12] , [13] , [14] or modulation [15] , [16] , [17] , [18] of conductive channels, tens or hundreds of nanometres in diameter, driven by the drift/diffusion of oxygen vacancies are believed to play a key role in the mechanism. In case of the well-established Pt/TiO 2 /Pt memristor devices, the state variable w is the tunnel barrier width between a top electrode (TE) and the preformed conductive filament, which is modified by the ionic drift within a few nanometre-thick space charge layer. The shift of ions in such a confined space must immediately equilibrate and the relaxation between high-resistive state (HRS) and low-resistive state (LRS) terminates within a few microseconds [16] , [19] , [20] . In principle, mixed ionic electronic conductors (MIEC) sandwiched by two blocking electrodes may show non-filamentary resistive switching, if the ions are uniformly conductive throughout the film bulk, even at room temperature, since the homogeneous migration of ions will modify the electronic carrier distribution across the conductor, and thus its bulk resistivity [3] , [21] , [22] , [23] . The bulk diffusion of dopants may require longer decay times and larger changes of bulk states until equilibrium than the ionic motion in a confined space. The suggested time dependency and number of resistance states in non-filamentary resistive switches are quite different from those in filamentary devices [5] , [7] , [24] , [25] . However, there are only very few well-known bulk memristive systems [25] , [26] , [27] , [28] , since the bulk ionic conductivity of MIECs is usually very low near room temperature. Furthermore, the direct evidence for the bulk state function of the switching system is still missing. Hence, it is a great challenge for material scientists to establish a non-filamentary-type MIEC memristor based on the efficient, bulk ion conduction at low temperatures. Herein, we demonstrate the homogeneous resistive switching in mixed oxide ion electron-conducting, amorphous gallium oxide thin films, a -GaO x , with the main state function being the time-dependent oxygen concentration profile across the film. The film possesses nonlinear, dynamical switching behaviour as is observed in the mathematically derived memristor model [2] , [3] , [21] , in which the I-V responses can be varied from a continuous counter figure-eight loop at high frequencies to a quasi-abrupt, triangle-like switching loop at lower frequencies, as depending on the bias history. This is the first report of the efficient oxide ion conductivity of an amorphous main-group oxide thin film at room temperature, perhaps opening up a new route to obtain dynamical, homogeneous switching memristor systems. The main objective of this study is to demonstrate the basic working principle of the homogeneous GaO x switching device, while technical characterization of the device is beyond the scope of this manuscript. Resistive switching behaviour Previously, we reported on the synthesis of highly nonstoichiometric, amorphous gallium oxide, a -GaO x ( x ~1.1), by a pulsed laser deposition (PLD) [29] . This oxide is—due to its high gallium excess—a heavily self-doped, n -type semiconductor [29] . Recently, several authors reported that a -GaO x thin films with Pt as TE and ITO or TiN as bottom electrode (BE) reveal a counter figure-eight hysteretic loop in their I-V characteristics [30] , [31] . They proposed a filamentary switching mechanism, similar to that introduced for TiO x , to explain GaO x switching [30] , [31] , [32] . However, there are qualitative differences in the memristive behaviour between GaO x and TiO x , as will be shown below. Thus, we propose a non-filamentary resistive switching mechanism for GaO x that is consistent with both the structure of the films and the observed switching dynamics. We first conducted a systematic study of the I-V characteristics by changing the film thicknesses, the voltage-sweep rates and the temperatures. For this purpose, we fabricated a film device of Pt-TE(100 nm)/GaO x /ITO-BE(40 nm) by depositing amorphous GaO x ( x ~1.1) films by PLD at the same conditions as described in our previous report [29] . The chemical composition was checked by using scanning transmission electron microscope equipped with energy dispersive X-ray spectrometer (STEM-EDX). A typical I-V curve for a 90-nm-thick film is shown in Fig. 1a . The pristine GaO x film clearly reveals a pinched hysteretic loop with counter figure-eight polarity as sweeping the voltage at the TE in the way of 0→+2→0→−2→0 V, indicating memristive behaviour of the film. A positive voltage (about +1.7 V) gradually increases the resistance so as to SET the film from the LRS to the HRS, and with negative bias (−2 V) the film is RESET to the LRS. This bipolar behaviour is stationary after the 1st sweep cycle, revealing that the pristine, homogeneous state (corresponding to the as-prepared film) is not recovered after the 1st cycle. We emphasize that the GaO x device does not require any electrical-forming process in contrast to TiO x -based devices where forming of filaments is a prerequisite [9] , [33] . This is a great advantage because the device reliability is independent on the reproducibility of the microstructural filament formation. 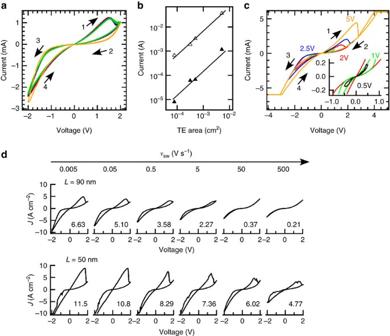Figure 1: Bipolar resistive switching of Pt(TE)/a-GaOx/ITO(BE) devices. (a)I-Vcharacteristics of a 90-nma-GaOxfilm during a 30-times voltage-sweep cycle of 0→+2→−2→0 V at a sweep ratevsw=0.05 V s−1and a temperature of 25 °C. The curves measured with TE diameter=200 μm and BE area=1 × 1 cm2for the 1st sweeping cycle (yellow), 2–10th cycles (red), 11–20th cycles (blue) and 20–30th cycles (green). The numbered arrows indicate the direction of the switching cycles (counter figure-eight loops). (b) TE area scaling of the current of LRS at −1.7 V (white triangles) and HRS at +1.7 V (black triangles). The solid lines for both plots show linear scaling with a slope of 1. (c)I-Vcharacteristics of 90 nm films measured atvswof 0.05 V s−1with various bias amplitudes. (d) Variable hystereticI-Vloops ofa-GaO1.1thin films with thickness of 50 and 90 nm, measured at 25 °C with various voltage-sweep ratesvswin the range of 0.005–500 V s−1. The numbers in each graph denote the hysteretic area (V A cm−2) of the loop.a-GaOxthin films can reveal non-hysteresis curves, counter figure-eight loops, triangular loops and quasi-abrupt switching-like loops as depending onvsw. Figure 1: Bipolar resistive switching of Pt(TE)/ a -GaO x /ITO(BE) devices. ( a ) I-V characteristics of a 90-nm a -GaO x film during a 30-times voltage-sweep cycle of 0→+2→−2→0 V at a sweep rate v sw =0.05 V s −1 and a temperature of 25 °C. The curves measured with TE diameter=200 μm and BE area=1 × 1 cm 2 for the 1st sweeping cycle (yellow), 2–10th cycles (red), 11–20th cycles (blue) and 20–30th cycles (green). The numbered arrows indicate the direction of the switching cycles (counter figure-eight loops). ( b ) TE area scaling of the current of LRS at −1.7 V (white triangles) and HRS at +1.7 V (black triangles). The solid lines for both plots show linear scaling with a slope of 1. ( c ) I-V characteristics of 90 nm films measured at v sw of 0.05 V s −1 with various bias amplitudes. ( d ) Variable hysteretic I-V loops of a -GaO 1.1 thin films with thickness of 50 and 90 nm, measured at 25 °C with various voltage-sweep rates v sw in the range of 0.005–500 V s −1 . The numbers in each graph denote the hysteretic area (V A cm −2 ) of the loop. a -GaO x thin films can reveal non-hysteresis curves, counter figure-eight loops, triangular loops and quasi-abrupt switching-like loops as depending on v sw . Full size image The homogeneous resistive switching mechanism is clearly demonstrated by two experimental findings shown in Fig. 1b,d . First, the current levels of our a -GaO x device linearly scale with the TE area ( Fig. 1b ; Supplementary Fig. 1 ). Second, we observe the wide variety of hysteretic shapes in the I-V curves, depending on the voltage-sweep rate ν sw and the film thickness L ( Fig. 1d ) The films reveal counter figure-eight loops, triangular loops, quasi-abrupt switching like loops and even non-hysteretic I-V curves. The hysteretic area in the I-V curves increases with decreasing film thickness and decreases with increasing voltage-sweep rate. Both observations are supportive for the homogeneous resistive switching mechanism triggered by bulk ion conduction and rule out a filamentary mechanism: First, as shown in Supplementary Fig. 1 the current density at the TE is independent on the TE area. Second, when the film thickness and/or the voltage-sweep rate increases no appreciable polarization of the ions can build up during one sweep cycle, and thus the hysteretic area decreases. Once the hysteretic area becomes very small, for example, in the 90-nm-thick film at high sweep rates, a nonlinear I-V curve is observed. This is probably due to the tunnelling nature of the interface between the high work function Pt electrode (5.6 eV (ref. 34 )) and the n -type gallium oxide [29] . Higher bias amplitudes also result in the transformation of the hysteretic loop in the anodic region from an ellipsoidal loop to a triangular one ( Fig. 1c ). Finally, we emphasize that all changes of the I-V curves shown in Fig. 1c,d are completely reversible (see Supplementary Fig. 2 ), showing that the films do not experience irreversible changes during switching. The complete series of I-V curves as function of film thickness, voltage-sweep rate and temperature as well is given in Supplementary Fig. 3 . 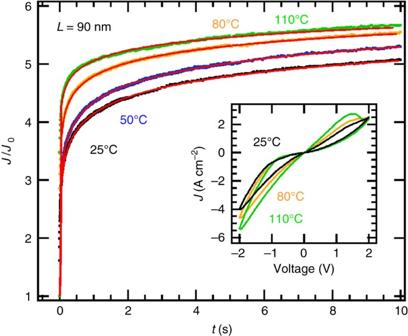Figure 2: Current transients ofa-GaOxfilms during resistive switching from HRS to LRS. Current transients of 90-nm-thick pristine films after applying a bias of −1.7 V to the TE att=0. The coloured dots are the measured values, and the red lines are the fits by a stretched exponential function,J/J0=Aexp{−(t/τ)β}, with fitting parameters of pre-exponential factorA, relaxation timeτ(s) and Kohlrausch stretching exponentβ(for details see main text). Inset: temperature dependence of theI-Vcharacteristics of 90-nm-thick films, measured atvsw=0.5 V− s−1. Best fitting for the 90 nm films at 25, 50, 80 and 110 °C was obtained with a set of parameters (A,τ,β)=(10.1, 0.24, 0.88), (9.4, 0.20, 0.88), (9.8, 0.057, 0.90) and (10.6, 0.011, 0.93), respectively. Figure 2 shows the current transient when a constant −1.7 V bias is suddenly applied on the pristine film at t =0. The negative current exponentially increases with increasing the bias duration, indicating that the resistance state of the pristine film decays exponentially to the LRS by cathodic polarization. The relaxation of the 90-nm-thick film apparently becomes faster with elevating temperature. The relaxation curves at each temperature can be described well by a stretched exponential relaxation function, which is represented by exp{−( τ / t ) β }.This result discloses that the resistive switching of a -GaO x is triggered by ion conduction and redistribution within its glassy matrix. The stretched exponential relaxation originates from the wide distribution of activation energies for ion conduction and the associated wide range of relaxation times among different relaxation processes in a disordered system [35] , [36] , [37] , [38] . Ion conductivity relaxation of many oxide glasses obeys this function because the structural inhomogeneity provides widely distributed activation energies for site-to-site hopping [36] , [37] , [38] . Here the Kohlrausch stretching exponent β ranging from 0 to 1 gives the correlation between the activation energy of ion conductivity E a * and average microscopic energy barrier E a impeding the ion movement between sites as defined by E a = β E a * (refs 36 , 37 , 38 ), and the relaxation time τ is proportional to ε 0 ε s σ dc −1 with ε 0 as permittivity of vacuum, ε s dielectric constant of the glass and σ dc its ion conductivity [36] . Empirically, it has been known that higher conductivity gives lower β and τ (refs 36 , 37 ). For cation conducting glasses with σ dc of ~10 −4 S cm −1 , β and τ are about 0.6 (ref. 38) [38] and about 10 ns (ref. 37 ), respectively. The fitting for the 90-nm-thick film gives β of about 0.9 and τ of >0.01 s at each temperature, revealing that the oxide ion conduction is rather low at the measured temperature range, as necessary for long retention times. The Arrhenius plot of τ yields an activation energy of E a *=0.5 eV for the ion conductivity ( Supplementary Fig. 4 ). As the ion conductivity increases with increasing temperature, the hysteretic loop of the I-V characteristics is clearly enlarged (inset of Fig. 2 ). Figure 2: Current transients of a -GaO x films during resistive switching from HRS to LRS. Current transients of 90-nm-thick pristine films after applying a bias of −1.7 V to the TE at t =0. The coloured dots are the measured values, and the red lines are the fits by a stretched exponential function, J / J 0 = A exp{−( t /τ) β }, with fitting parameters of pre-exponential factor A , relaxation time τ (s) and Kohlrausch stretching exponent β (for details see main text). Inset: temperature dependence of the I-V characteristics of 90-nm-thick films, measured at v sw =0.5 V− s −1 . Best fitting for the 90 nm films at 25, 50, 80 and 110 °C was obtained with a set of parameters ( A , τ , β )=(10.1, 0.24, 0.88), (9.4, 0.20, 0.88), (9.8, 0.057, 0.90) and (10.6, 0.011, 0.93), respectively. Full size image Valence change by homogeneous oxide ion migration As a consequence of the electrochemical polarization of the GaO x films the Ga valence must change as a function of the applied bias. In order to identify the Ga valence states in the HRS and the LRS micrometre probe X-ray photoelectron spectroscopy (μ-XPS) was performed on the bare surface of polarized films after removing the TE ( Fig. 3a ). Ga 3D photoemission electron microscopy (PEEM) images taken at a binding energy of 20.6 eV ( Fig. 3b ) clearly differentiate between the HRS film within the TE mark area (bright) and the pristine surface area (grey), thus indicating differences in the Ga valence states between the polarized and the unpolarized regions. The corresponding spectra (red and blue lines in the inset of Fig. 3b ) more clearly demonstrate that the Ga valence state changes by polarization. 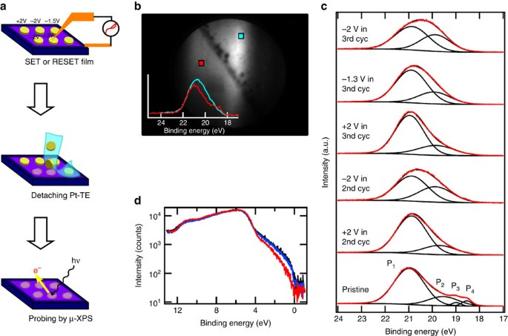Figure 3: Homogeneous Ga valence state change through resistive switching ofa-GaOxdevice. (a) Procedure to prepare the barea-GaOxsurface after polarization to the HRS or LRS. After polarization, UV set epoxy resin was pasted on the TE, and the TE was removed by scratching off the epoxy resin. (b) Photoemission electron microscopy (PEEM) image in the Ga 3d binding energy region, measured at the border of the pristine surface (bright grey region with red square) and the bare surface of HR film under the +2 V-biased TE mark (diameter=200 μm) (dark grey region with blue square). The black line along the border is due to segregation of contaminants such as Pt and resin residues. Inset: XPS spectra were reconstructed from the PEEM images at the red point within the pristine surface area (red line) and at the blue point within the polarized surface area (blue line). (c) μ-XPS in the Ga 3d binding energy region measured on the pristine surface and at marks of the TE polarized at different voltages during the 2nd and 3rd sweep cycle. In the polarized films, the measured spectrum (red dots) can be described well by two peaks (black line) corresponding to Ga3+(P1) and Ga+(P2), that is, Ga is highly reduced. A couple of peaks corresponding to metallic Ga0(P3and P4) are involved only in the unpolarized, pristine film. Molar ratios of Ga3+/Ga+are 0.16/0.84 at 2 V and 0.52/0.48 at −2 V in the 2nd sweep cycle and 0.19/0.81 at 2 V, 0.28/0.71 at −1.3 V and 0.50/0.50 at −2 V in the 3rd sweep cycle, as calculated by peak fitting analysis. (d) Near-Fermi edge spectra of a-GaOxfilm: pristine (black), HRS (at +2 V) (red) and LRS (at −2 V) (blue). The density of states near the top of the valence band is variable by negative or positive biasing. Figure 3c shows the μ-XPS spectra collected on the pristine and polarized film surfaces, respectively. The pristine film exhibits three different Ga valence states; a strong peak at 20.7 eV (P 1 ) is assigned to the oxide (Ga 3+ ) [39] state, a peak at around 19.6 eV (P 2 ) to the suboxide (Ga + ) [39] , [40] state and a pair of small peaks at 18.7 (P 3 ) and 18.2 eV (P 4 ) can be assigned to the metal (Ga 0 ) state (by comparing with a GaCo alloy reference sample, Supplementary Fig. 5 ). The average valence state of Ga in the pristine film is calculated to be +2.3 ( Table 1 ), in good agreement with the value +2.2 that is calculated from the composition of the film, GaO 1.1 , obtained by STEM-EDX. Figure 3: Homogeneous Ga valence state change through resistive switching of a -GaO x device. ( a ) Procedure to prepare the bare a -GaO x surface after polarization to the HRS or LRS. After polarization, UV set epoxy resin was pasted on the TE, and the TE was removed by scratching off the epoxy resin. ( b ) Photoemission electron microscopy (PEEM) image in the Ga 3d binding energy region, measured at the border of the pristine surface (bright grey region with red square) and the bare surface of HR film under the +2 V-biased TE mark (diameter=200 μm) (dark grey region with blue square). The black line along the border is due to segregation of contaminants such as Pt and resin residues. Inset: XPS spectra were reconstructed from the PEEM images at the red point within the pristine surface area (red line) and at the blue point within the polarized surface area (blue line). ( c ) μ-XPS in the Ga 3d binding energy region measured on the pristine surface and at marks of the TE polarized at different voltages during the 2nd and 3rd sweep cycle. In the polarized films, the measured spectrum (red dots) can be described well by two peaks (black line) corresponding to Ga 3+ (P 1 ) and Ga + (P 2 ), that is, Ga is highly reduced. A couple of peaks corresponding to metallic Ga 0 (P 3 and P 4 ) are involved only in the unpolarized, pristine film. Molar ratios of Ga 3+ /Ga + are 0.16/0.84 at 2 V and 0.52/0.48 at −2 V in the 2nd sweep cycle and 0.19/0.81 at 2 V, 0.28/0.71 at −1.3 V and 0.50/0.50 at −2 V in the 3rd sweep cycle, as calculated by peak fitting analysis. ( d ) Near-Fermi edge spectra of a-GaO x film: pristine (black), HRS (at +2 V) (red) and LRS (at −2 V) (blue). The density of states near the top of the valence band is variable by negative or positive biasing. Full size image Table 1 Summary of Ga 3d μ -XPS on polarized a -GaO x films. Full size table It appears that the Ga valence state within the whole TE mark area is homogeneously switched by anodic or cathodic polarization. The valence state of Ga is variable between Ga 3+ and Ga + and the metallic state does not evolve again after the 1st sweep cycle. Therefore, the different behaviour in the 1st voltage-sweep cycle (see Fig. 1a ) is due to the oxidation of Ga 0 to Ga + and Ga 3+ . In the 2nd sweep cycle, when sweeping the voltage to +2 V (SET the film to HRS) >80% of Ga exists in the highest oxidation state (Ga 3+ ) as calculated from the P 1 /P 2 peak area ratio, and so the average oxidation state of Ga increases from +2.3 in the pristine film to +2.7 ( Table 1 ). RESET to the LRS by negative biasing (−2 V) reduces GaO x (with about 50% of Ga in the suboxide state Ga + ) so as to complete the Ga redox cycle. These results strongly indicate that positive or negative bias on the TE homogeneously oxidizes or reduces the GaO x underlayer, respectively, by migration of oxygen ions (or oxygen vacancies) towards or away from the TE. This must cause the modification of the donor density in the underlayer since oxygen vacancies act as donors in GaO x (ref. 29 ). In fact, the near-Fermi edge spectra in Fig. 3d show that the density of states near the VB edge is also variable throughout the redox cycle of the film; that of a pristine film is decreased by oxidation at +2 V, but is increased again to the similar level as that of the pristine film by reduction at −2 V. Such a Ga redox cycle is clearly reproducible in the 3rd sweep cycle. Furthermore, the molar ratio of Ga + /Ga 3+ continuously increases in proportion to the negative bias amplitude as 0.3/0.7 at −1.3 V and 0.5/0.5 at −2 V ( Fig. 3d ), indicating that the oxidation state of GaO x is continuously variable. Finally, we emphasize that it would be impossible to detect the observed Ga valency changes in the polarized regions for filamentary switching, as the cross-section area of one or a few filaments would be by far too small to cause changes in the XPS signals originating from the large cross-section area of the exciting X-ray beam ( Supplementary Fig. 6 ). 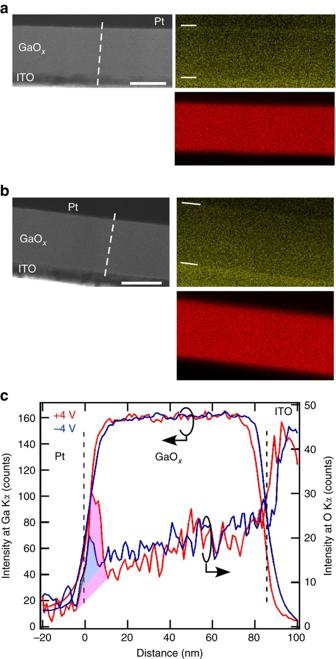Figure 4: Cross-sectional electron microscopy of Pt/a-GaOx(90 nm)/ITO devices after switching to HRS and LRS. (a) STEM images and the corresponding EDX elemental mapping of O (yellow) and Ga (red) of the HRS film after polarization at +4 V during the 3rd −4 V→+4 V voltage-sweep cycle atvswof 0.5 V s−1. (b) STEM images of the −4 V-biased film in LRS. The scale bars in (aandb) are 40 nm. The solid white lines in the O EDX mapping images are a guide to the eye for the boundaries of the GaOxfilm. (c) EDX line profiles of O and Ga scanned from the Pt to the ITO side along the white dashed lines in the STEM images inaandb. The line profiles of O are obtained by subtracting the background noise determined from an Al standard sample. The EDX line profiles apparently show the enrichment of O near the TE/film boundary (magenta-filled peak area) by anodic polarization and the decrease of O at the BE/film boundary (cyan-filled peak area) by cathodic polarization. In contrast, the Ga line profile remains flat, independent of anodic or cathodic polarization. Figure 4 shows the STEM-EDX images of a cross-section of a 90-nm film that was polarized to a cathodic or anodic direction. Even after the polarization to +4 V or −4 V, no heterogeneous microstructure consisting of crystalline domains or metallic filaments could be found in >10 examined specimens. EDX elemental mapping images clearly elucidate that oxygen is segregated within the film near the TE/film boundary by polarization to +4 V, but the segregation is diminished after polarization to −4 V ( Fig. 4a,b ). Furthermore, the interfacial layer is uniformly enriched and depleted by oxygen according to the bias direction, revealing the non-filamentary switching behaviour. Figure 4c shows the oxygen and gallium line profiles across the films. The films polarized at +4 V are comprised of three O-concentration regions: an O-enriched region near the TE/film boundary within a thin, about 10-nm-wide layer (red-filled area in Fig. 4c ), a region with low O-concentration at intermediate depths ranging from 10 to 30 nm and a middle O-concentration region in the depth range of 40 to 90 nm. In contrast, the Ga profile is kept flat throughout the film. When subsequently negative bias is applied to the TE, the O-enrichment near the TE/film boundary is decreased (compare red- and blue-filled areas), and the concentration in the intermediate depth region is slightly increased. This observation clearly shows that the resistive switching of GaO x is caused by mobile oxygen ions and the modulation of the oxygen concentration profile, as a result of electrochemical polarization due to the applied voltage. Figure 4: Cross-sectional electron microscopy of Pt/ a -GaO x (90 nm)/ITO devices after switching to HRS and LRS. ( a ) STEM images and the corresponding EDX elemental mapping of O (yellow) and Ga (red) of the HRS film after polarization at +4 V during the 3rd −4 V→+4 V voltage-sweep cycle at v sw of 0.5 V s −1 . ( b ) STEM images of the −4 V-biased film in LRS. The scale bars in ( a and b ) are 40 nm. The solid white lines in the O EDX mapping images are a guide to the eye for the boundaries of the GaO x film. ( c ) EDX line profiles of O and Ga scanned from the Pt to the ITO side along the white dashed lines in the STEM images in a and b . The line profiles of O are obtained by subtracting the background noise determined from an Al standard sample. The EDX line profiles apparently show the enrichment of O near the TE/film boundary (magenta-filled peak area) by anodic polarization and the decrease of O at the BE/film boundary (cyan-filled peak area) by cathodic polarization. In contrast, the Ga line profile remains flat, independent of anodic or cathodic polarization. Full size image Numerical simulation by mixed oxide ion electron conduction The above experimental findings unambiguously demonstrate that in our GaO x films a whole oxide layer below the TE is homogeneously oxidized/reduced. These features do not adapt to the filamentary switching driven by locally occurring ion migration. In addition, the STEM-EDX measurements disclose that the bulk oxide ion conductivity is essential for the resistive switching of GaO x . Here, we provide a physical model for the homogeneous switching based on mixed oxide ion electron conduction under an applied electrochemical potential gradient. This model assumes that the resistive switching is due to the modulation of the carrier concentration profiles in the amorphous n -type semiconductor by redistribution of the oxygen vacancy donor. As our model calculations can reproduce the experimentally observed I-V curves very well, we believe that the interfacial effect, that is, the Schottky barrier at the Pt/GaO x interface is of minor importance in GaO x , and thus it is omitted in our model for simplification. In our simulations the relations of the dimensions of the TE and the BE are similar to those of the test samples (the former with a diameter of 200 μm and the latter with an area of 1 × 1 cm 2 ), which enables calculating the effect of in-plane diffusion according to the concentration gradients. The detailed explanation of the model and the simulation procedure are given in the Methods section. The simulation semiquantitatively replicates the experimentally observed I-V characteristics, exhibiting an asymmetric pinched loop in a bipolar manner (counter figure-eight loop) by switching from LRS to HRS in the anodic region and from HRS to LRS in the cathodic region. Typical simulation results are shown for the 2nd sweep cycle of a 90-nm-thick film in Fig. 5 . Best agreement between experiment and simulation was obtained with a vacancy mobility μ V =7 × 10 −19 m 2 V −1 s −1 . All other parameters were fixed as specified in the Methods section. In addition to the I-V curve, the calculated oxygen vacancy profiles across the film and the corresponding electronic conductivities are shown at different stages of electrochemical polarization. The electronic conductivity of amorphous semiconductors tends to increase exponentially with an increasing vacancy concentration (donor concentration), since the mobile carrier concentration is related to an energy gap between the Fermi level and mobility edge [41] . At the beginning of the 2nd sweep cycle, that is, for small anodic voltages (point 1 in Fig. 5 ) there is still an inhomogeneous distribution of oxygen vacancies due to the preceding cathodic polarization in the 1st sweep cycle. When the bias is swept to +1.5 V (point 2 in Fig. 5 ) the oxygen vacancy concentration near the TE/film boundary decreases, but as polarization is still relatively small the film remains in the LRS. At point 3 in Fig. 5 the depletion of oxygen vacancies near the TE is already stronger, and due to the exponential dependence of the electronic conductivity on the vacancy concentration the transition to the HRS starts. Point 4 in Fig. 5 is typical for the HRS. Compared with point 2 (LRS) the vacancy concentration near the TE has decreased only by several per cent, however, the electronic conductivity has decreased by a factor of 6, producing a HR region near the TE. For cathodic polarization, the depleted region is filled again with oxygen vacancies (point 5) resulting in the transition from HRS to LRS and at point 6 the initial configuration in point 1 is nearly recovered. As the applied voltage will drop mainly within the very high-resistive region formed near the TE, the shift of oxygen vacancies extensively occurs within a few 10-nm-wide layer near the TE/film interface. This feature is in agreement with the observations that the oxygen concentration near the TE is increased/decreased by charge/discharge of oxide ions in the neighbouring, intermediate depth region ( Fig. 4c ). 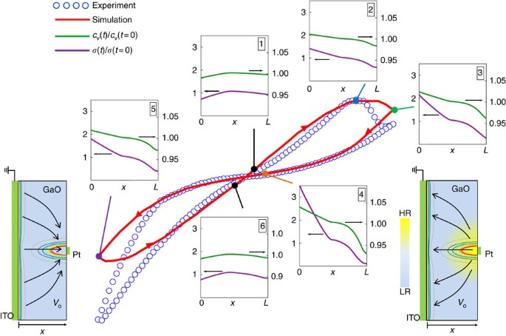Figure 5: Simulation ofa-GaOxresistive switching with a model based on drift diffusion of oxygen vacancy donors under electrochemical potentials. Observed (blue circles) and calculated (red line)I-Vcurves of the 2nd sweep cycle of a 90-nm-thicka-GaOxfilm at a sweep rate of 0.05 V s−1andT=25 °C. Best agreement between experiment and simulation was obtained with a vacancy mobilityμV=7 × 10−19m2V−1s−1. All other parameters were fixed as specified in the Methods section. Also shown are the calculated concentration profiles of oxygen vacancies,cV, and the corresponding electronic conductivitiesσe(normalized by their respective initial values) across the film at 0.1 V (point 1, black), 1.5 V (point 2, blue), 2 V (point 3, green), 0.2 V (point 4, orange), −2 V (point 5, purple) and −0.1 V (point 6, black).xis the distance from the BE/film interface. The right and left counter images show schematically the electrochemical equipotential lines at points 4 (HRS) and 5 (LRS), respectively, and the schematic representation of the switching between HRS and LRS due to the flux of oxygen vacancies (VO) under the applied electrochemical potential gradients. At point 4, a region beneath the TE (yellow region) is strongly depleted by oxygen vacancies, and due to the charge balancece=2cVit is also depleted by electrons causing the HRS. At point 5 the depleted region is partly refilled by oxygen vacancies and electrons (blue region), resulting in the LRS. Details of the calculation can be found in the Methods section. Figure 5: Simulation of a -GaO x resistive switching with a model based on drift diffusion of oxygen vacancy donors under electrochemical potentials. Observed (blue circles) and calculated (red line) I-V curves of the 2nd sweep cycle of a 90-nm-thick a -GaO x film at a sweep rate of 0.05 V s −1 and T =25 °C. Best agreement between experiment and simulation was obtained with a vacancy mobility μ V =7 × 10 −19 m 2 V −1 s −1 . All other parameters were fixed as specified in the Methods section. Also shown are the calculated concentration profiles of oxygen vacancies, c V , and the corresponding electronic conductivities σ e (normalized by their respective initial values) across the film at 0.1 V (point 1, black), 1.5 V (point 2, blue), 2 V (point 3, green), 0.2 V (point 4, orange), −2 V (point 5, purple) and −0.1 V (point 6, black). x is the distance from the BE/film interface. The right and left counter images show schematically the electrochemical equipotential lines at points 4 (HRS) and 5 (LRS), respectively, and the schematic representation of the switching between HRS and LRS due to the flux of oxygen vacancies ( V O ) under the applied electrochemical potential gradients. At point 4, a region beneath the TE (yellow region) is strongly depleted by oxygen vacancies, and due to the charge balance c e =2 c V it is also depleted by electrons causing the HRS. At point 5 the depleted region is partly refilled by oxygen vacancies and electrons (blue region), resulting in the LRS. Details of the calculation can be found in the Methods section. Full size image The equipotential lines at +0.2 and −2 V bias on the small area TE are shown schematically in the inset of Fig. 5 , indicating that the large bias is applied in the vicinity of the TE, but the potential tends to be flat and to extend transversally over a wide area close to the large area BE. The transversal oxide ion diffusion occurs in the interior of the film according to the in-plane oxygen concentration gradients initiated by drift, modifying the in-plane donor distribution. Therefore, the current flux lines are widely broadened near the BE. These results indicate that the device configuration has an important role to tune the switching dynamics in bulk diffusion-based memristors. Recently, Meyer et al. [28] reported a resistive switching memory utilizing oxide ion migration in a conductive metal-oxide (CMOx) thin film. The device consisting of a stack of a CMOx film and a few nanometre-thick tunnel oxide (TO) layer reveals homogeneous resistive switching due to modulating the tunnel barrier height by the oxygen exchange between CMOx and TO. The devices switch very fast, typically on a microsecond time scale because the distance oxide ions travel during switching events is on an atomic scale. Our a -GaO x device does not need the interfacial TO layer for switching and, furthermore, the current is controlled by bulk resistance states rather than interfacial states. Therefore, it is easily expected that switching events and relaxation of resistance states of our a -GaO x device require longer periods of time than in the CMOx device because the oxygen bulk diffusion distance is larger than that of the interfacial exchange. In this study, we demonstrated that homogeneous resistive switching occurs in mixed oxide ion electron-conducting, amorphous gallium oxide thin films. The donor distribution is modified by the forward drift motion of oxygen vacancies by the external field and the compensation of the preceding drift by diffusion along the oxygen concentration gradient. Hence, the bulk oxygen concentration profile across the film takes the role of the internal state variable in the a -GaO x device. This bulk drift-diffusion mechanism gives rise to a clear response transient compared with filamentary mechanism devices, which tend to show a quasi-abrupt transition between HRS and LRS because of the relaxation time of the order of sub-microseconds [4] , [16] , [20] . In contrast, homogeneous resistive switching of GaO x proceeds gradually during the bias duration in the range from sub-milliseconds to seconds. Thus, the time dependency provides the reversible transformation of the I-V hysteretic loop as is observed in the mathematically derived memristor model. These features can be attributed to the time-dependent internal state function, which is controlled not only by the external field but also by the in- and out-of plane electrochemical potential gradients. Apparently, the resistance state of the a -GaO x semiconductor can be efficiently tuned even with low oxide ion conduction at room temperature. Accordingly, it is concluded that amorphous oxide semiconductors with a mixed oxide ion electron conductivity have the potential for a dynamical memristor system realizing multilevel states of resistance and a large on/off current ratio due to the continuous tunability of the internal state variable. To develop feasible homogeneous resistive switching devices for future neuromorphic application [4] , [6] , [24] , mixed ion electron-conducting amorphous oxides may be very beneficial. Unfortunately, the established oxide ion-conducting glasses have been still missing [42] , and so the mechanism of oxide ion conduction in glasses remained unclear. Meanwhile, the preceding results strongly suggest that the low-temperature oxide ion diffusivity of a -GaO x film must be related to its local coordination environment and interstitial space of the highly oxygen-deficient Ga-O glass network. The current findings possess an opportunity to investigate the memristive switching in highly nonstoichiometric metal oxides whose stoichiometric phase is known to be a poor ion conductor. Preparation and characterization Highly nonstoichiometric amorphous gallium oxide thin films, a -GaO x , were deposited on a substrate by PLD with a KrF excimer laser ( λ =248 nm, pulse energy=300 mJ, sequence=10 Hz, Lambda Physik) [29] . ITO-coated SiO 2 glass (Aldrich) was used as a BE substrate. Sintered pellets of Ga 2 O 3 (Alfa Aesar, 99.999%) were prepared as a PLD target. The laser-evaporated species were deposited onto the substrates at 300 K in atmospheres of pure argon at a pressure of 30 mTorr. Current–voltage ( I-V ) characteristics were measured using a Keithley 2612A source metre. The Pt top electrode (200 μmφ, 50 nm thickness) was sputter-deposited on the film through a metal shadow mask. All measurements were conducted on a custom-made probe station equipped with a plate heater in the glove box under a dry argon atmosphere. STEM-EDX analysis was conducted with Hitachi HD-2200 scanning transmission electron microscope. The line profiles of oxygen and gallium were corrected by subtracting the background noises determined from the Al standard sample. The ultrathin sample was prepared by the combination of a focused ion beam (Hitachi FB-2100) and Ar ion milling (Gatan 691). Synchrotron X-ray photoemission electron microscope Photoemission electron microscopy and μ-XPS measurements were performed at the NanoESCA beamline at synchrotron facility Elettra [43] . A Pt/GaO x /ITO device with a-GaO x layer of 50 nm thickness and Pt TE of 200 μm diameter was used as a specimen for NanoESCA. The TE was cathodically or anodically polarized by sweeping the voltage in the range of −2 to +2 V at a sweep rate of 0.005 V s −1 in order to create a HRS or LRS film. After sweeping, ultraviolet (UV)-set resin (three-bond 3000) was applied onto the TE through a microsyringe and polymerized by UV irradiation with a Hg lamp. The resin was slipped off from the surface by scratching it with a sharp tweezer, and thus the TE was detached from the film so as to form the bare surface of the polarized GaO x film. Most of these operations were performed under the optical microscope. Numerical simulation The flux J i of charged species i (electrons and ions) can be expressed by where F , z i , σ i and η i are the Faraday constant, formal charge number, partial conductivity and electrochemical potential of species i, respectively. In the GaO thin film, the ionic species could be gallium ions being mobile as gallium interstitials, , or oxygen ions being mobile via oxygen vacancies, (ref. 26 ). Here, we assumed as mobile charge carriers electrons, e, and oxygen ions (being mobile via ) in accordance with the STEM-EDX results. We have simulated the memristor behaviour of the GaO thin film device numerically by using the 3D finite element method (Comsol Multiphysics). For the oxygen vacancies with concentration c V and partial conductivity σ V =2 Fμ V c V ( μ V =mobility) we solved the continuity equation with the following initial and boundary conditions The driving force for the vacancy flux is given by the gradient of the electrochemical potential of oxygen ions (see equation 1). Using the chemical equilibria for the quasi-chemical reactions O 2− ↔O+2e − and (Kroeger–Vink notation) the driving force can be written as: where x V = V m c V and x e = V m c e are the molar fractions of vacancies and electrons, c V and c e are their concentrations and V m is the molar volume of GaO. In equation (5) we have assumed for the sake of simplicity ideal behaviour of vacancies and electrons, and we have used the local charge neutrality within the film volume: The flux of electrons is determined by the electronic conductivity σ e and the gradient of the electrochemical potential of electrons η e (see equation (1)). Highly nonstoichiometric, amorphous GaO can be considered to be a heavily self-doped n -type semiconductor [26] . In such a highly disordered system, the mobile carrier concentration is not equivalent to the total electron concentration c e , because the electronic states below the mobility edge E m tend to be localized, and according to Mott [41] the electronic conductivity is given by where Δ E is the difference between the mobility edge E m and the Fermi energy E F . Experiments and theoretical calculations [29] for amorphous GaO have shown that Δ E decreases linearly with increasing electron fraction x e = V m c e , that is, Δ E = A − B x e with A =1.165 eV and B =0.513 eV, and the pre-factor is given by σ 0 =2 × 10 3 S m −1 . Due to the local charge neutrality within the film volume (see equation (6)), the electronic conductivity shows a very strong, exponential dependence on the local vacancy concentration. As a consequence of the local charge neutrality (equation (6) the divergence of the electric current density must vanish within the bulk of the film: Equation (9) is the differential equation from which the electrochemical potential η e can be calculated that has to satisfy the following boundary conditions at the BE and TE: Here V ( t ) is the applied voltage. Equation (1, 2, 3, 4, 5, 6, 7, 8, 9, 10, 11) form the necessary and sufficient set of equations to calculate the vacancy concentration c V and the electrochemical potential of electrons η e as a function of position and time. From these quantities the fluxes J V and J e and finally the current density i as a function of the applied voltage V ( t ) can be calculated. A typical simulated I-V characteristic of a GaO thin film is shown in Fig. 5 . How to cite this article: Aoki, Y. et al. Bulk mixed ion electron conduction in amorphous gallium oxide causes memristive behaviour. Nat. Commun. 5:3473 doi: 10.1038/ncomms4473 (2014).